Genome of the red algaPorphyridium purpureum The limited knowledge we have about red algal genomes comes from the highly specialized extremophiles, Cyanidiophyceae. Here, we describe the first genome sequence from a mesophilic, unicellular red alga, Porphyridium purpureum . The 8,355 predicted genes in P. purpureum , hundreds of which are likely to be implicated in a history of horizontal gene transfer, reside in a genome of 19.7 Mbp with 235 spliceosomal introns. Analysis of light-harvesting complex proteins reveals a nuclear-encoded phycobiliprotein in the alga. We uncover a complex set of carbohydrate-active enzymes, identify the genes required for the methylerythritol phosphate pathway of isoprenoid biosynthesis, and find evidence of sexual reproduction. Analysis of the compact, function-rich genome of P. purpureum suggests that ancestral lineages of red algae acted as mediators of horizontal gene transfer between prokaryotes and photosynthetic eukaryotes, thereby significantly enriching genomes across the tree of photosynthetic life. The red algae (Rhodophyta) form a monophyletic lineage comprising around 6,100 known species and 14,000 that are estimated to exist [1] . These taxa lack both flagella and centrioles during their life cycle [2] . Rhodophytes include many unicellular mesophilic lineages, the extremophilic Cyanidiophyceae (for example, Cyanidioschyzon and Galdieria ) that live in hot springs such as in Yellowstone National Park, and economically important seaweeds such as Gracilaria and Pyropia (including Porphyra ) [3] that are sources of agar and nori , respectively. Two aspects of red algal evolution are of central importance to understanding the evolution of eukaryotic phytoplankton. The first is their membership in the foundational lineage of photosynthetic eukaryotes, the supergroup Plantae (red algae, glaucophytes and green algae plus plants (also known as Archaeplastida)), whose ancestor putatively captured the canonical cyanobacterium-derived plastid [4] , [5] . The second is the subsequent spread of this organelle through secondary endosymbiosis to a diverse array of photosynthetic lineages collectively referred to as ‘chromalveolates’ (for example, diatoms, haptophytes and dinoflagellates [6] , [7] ) that are dominant marine primary producers. For instance, red alga-derived plastids in diatoms are responsible for about 25–50% of organic carbon fixed annually in the world’s oceans [8] . Secondary endosymbiosis also resulted in endosymbiotic gene transfer [9] (EGT) that relocated hundreds of former red algal genes to the nucleus of photosynthetic chromalveolates. Despite their central role in phytoplankton evolution, the genetic inventory of a unicellular lineage that may have been related to the putative donor of the ‘red plastid’ in chromalveolates is yet to be described. Existing rhodophyte complete genome sequences are from the thermoacidophiles Cyanidioschyzon merolae [10] and Galdieria sulphuraria [11] that have highly specialized and reduced genomes (for example, 16.5 Mbp with 5,331 protein-coding genes in C. merolae [10] ) and from the red seaweed Chondrus crispus [12] . Here, we analyse the draft genome assembly from the unicellular, mesophilic red alga Porphyridium purpureum CCMP 1328 (referred to as P. cruentum in this culture collection) ( Fig. 1a ). This strain was isolated in 1957 from Eel Pond, Massachusetts and for this project was cultured in f/2 enriched seawater medium. We elucidate the role of horizontal gene transfer (HGT) in enriching the genome of P. purpureum and the extent of red algal gene sharing via EGT or HGT with chromalveolates and other taxa. We also analyse key aspects of red algal biology such as the evolution of proteins involved in light harvesting and metabolite transport and in starch, lipid and isoprenoid biosynthesis, and search for evidence of sexual reproduction in this species. 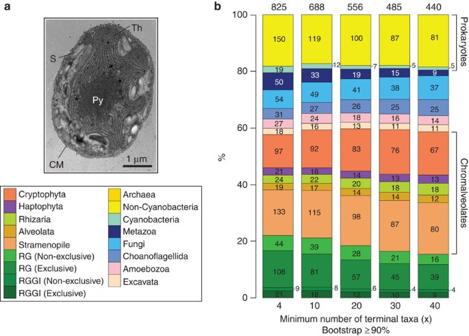Figure 1: Analysis of theP. purpureumgenome. (a) Transmission electron microscopy image of aP. purpureumcell showing the central pyrenoid (Py), cell membrane (CM), starch granules (S) and plastid thylakoids (Th). (b) Percentage of single protein RAxML trees (raw numbers shown in the bars) that support the monophyly ofP. purpureum(bootstrap ≥90%) solely with other Plantae members (exclusive), or in combination with non-Plantae taxa that interrupt this clade (non-exclusive). These latter groups of trees are primarily explained by red/green algal EGT into the nuclear genome of chromalveolates. For each of these algal lineages, the set of trees with different numbers of taxa (x) ≥4, ≥10, ≥20, ≥30 and ≥40 in a tree are shown. Each tree has ≥3 phyla. The Plantae-only groups are reds-greens-glaucophytes (RGGl) and reds-greens (RG). Figure 1: Analysis of the P. purpureum genome. ( a ) Transmission electron microscopy image of a P. purpureum cell showing the central pyrenoid (Py), cell membrane (CM), starch granules (S) and plastid thylakoids (Th). ( b ) Percentage of single protein RAxML trees (raw numbers shown in the bars) that support the monophyly of P. purpureum (bootstrap ≥90%) solely with other Plantae members (exclusive), or in combination with non-Plantae taxa that interrupt this clade (non-exclusive). These latter groups of trees are primarily explained by red/green algal EGT into the nuclear genome of chromalveolates. For each of these algal lineages, the set of trees with different numbers of taxa (x) ≥4, ≥10, ≥20, ≥30 and ≥40 in a tree are shown. Each tree has ≥3 phyla. The Plantae-only groups are reds-greens-glaucophytes (RGGl) and reds-greens (RG). Full size image Assembly and genome characteristics The P. purpureum nuclear genome, based on the total length of the assembled contigs, was estimated to be 19.7 Mbp in size. This genome is intron-poor with 235 spliceosomal introns present in the 8,355 gene models (that is, 2.8% of genes contain introns) predicted using mRNA-seq data (see Methods for details). In comparison, 0.5% of genes in C. merolae contain introns [13] . The mapping of 52 million genome sequence reads to the consensus assembly showed the presence of 26,383 single-nucleotide polymorphisms in contigs with average coverage >10 × . Of these single-nucleotide polymorphisms, 94.6% were represented by two variants with an average representation of 57.5 and 42.4% for each variant, suggesting that the P. purpureum strain we sequenced was diploid. Previous studies have suggested both haploidy [14] and diploidy in this genus with the presence of 8–10 chromosomes [15] . Other analyses of the genome are shown in Supplementary Fig. S1 , Supplementary Tables S1 and S2 , and described in the Supplementary Information . The assembled genome and cDNA contigs, gene models, gene annotations, phylogenomic output and other material are available at http://cyanophora.rutgers.edu/porphyridium/ . Analysis of gene transfer Phylogenomic analysis ( Supplementary Table S3 ) resulted in 5,996 maximum likelihood protein trees (that is, 71.8% of the 8,355 total predicted proteins). At the stringent bootstrap threshold of ≥90% (or at ≥70 and ≥50%; Supplementary Fig. S2 ; lists of sorted phylogenies in Supplementary Tables S4–S6 ), about 20% of the trees supported the monophyly of red algae and other Plantae either by themselves (exclusive) or including other taxa (non-exclusive) that could have gained the Plantae gene through EGT or HGT ( Fig. 1b ; and Methods section). At the bootstrap support threshold of ≥90%, we found 440–825 trees (7–14% of total trees; 5–10% of total 8,355 proteins) that show a strong association between red algae with one other lineage. As shown in Supplementary Fig. S2 , these numbers increase at the lower thresholds of ≥70% (766–1,310; 13–22% of total trees) and ≥50% (1,233–2,007; 21–33% of total trees). Of these trees (at bootstrap ≥90% in Fig. 1b ), ~40% showed sharing of red algal genes with different chromalveolate lineages either as nuclear genes or as cryptophyte nucleomorph-encoded [16] homologues (for example, 60S ribosomal protein L10A; contig 2315.2, Supplementary Data 1 ), and ~20% with prokaryote lineages. In an independent assessment of proteins in C. merolae , the corresponding proportion of prokaryote-associated red algal genes in this species is smaller (12%; Supplementary Fig. S3 ). The majority of the P. purpureum trees (>80% in the analysis based on a bootstrap threshold ≥90%) show an evolutionary history that is, however, too complicated (for example, poor resolution of clades or currently too few taxa in the trees) to interpret with confidence. Taking trees containing ≥3 phyla and ≥20 terminal taxa as an indicator (middle bar; Fig. 1b ), our results suggest that at least 453 genes (non-green portion; 5.4% of 8,355 proteins) in P. purpureum are impacted by E/HGT in their evolutionary history (773 genes at bootstrap ≥70%; 9.3% of 8,355). The complexity of these gene phylogenies is comparable to previous findings based on red algal transcriptome data [4] , [17] . Using a stringent criterion ( P ≤0.05 and false discovery rate ≤0.10), we observed no significant biases in the putative functions of P. purpureum proteins that are associated with non-Plantae taxa (non-green portion in Fig. 1b ) in comparison with the annotated functions across the whole data set ( Supplementary Fig. S4 ; Supplementary Tables S7–S9 ). Such functional biases were observed in an earlier study based solely on transcriptome data [18] . This discrepancy is likely explained by EST assembly artifacts in the earlier analysis that resulted in partial or mis-assemblies that inflated the total number of genes and their relative representation in the database. Nevertheless, among genes with phylogenies that show clear evidence of a common origin in Plantae, we found significant over-representation of gene ontology (GO) terms [19] related to reproductive and cell development ( Table 1 ), compared with the overall gene set (see Methods). This finding suggests that these genes are more likely to be vertically inherited within Plantae, or alternatively, that radiation/innovation of these genes occurred after the divergence of this supergoup. Table 1 Summary of over-represented gene ontology terms. Full size table Given the complex evolutionary history of red algal genes found using phylogenomics combined with potential issues associated with the interpretation of results from automated pipelines [20] , we conducted a manual analysis of a contig in our assembly to test the results regarding E/HGT. Contig 2035 (of size 91,179 bp) has average coverage of 623 × and encodes 42 genes, all with transcriptome evidence that show a paucity of spliceosomal introns ( Supplementary Fig. S5 ). This P. purpureum genome region encodes proteins with a diversity of evolutionary histories. For example, one eukaryotic gene (contig 2035b.35) shows the expected monophyly of the lineages red algae, plants, Fungi and Metazoa in the eukaryotic tree of life ( Fig. 2a ), whereas the neighbouring gene (contig 2035b.36), although also of eukaryotic provenance shows a reticulate history that involves Viridiplantae and chromalveolates ( Fig. 2b ). Other genes on contig 2035 are apparently of bacterial origin with one that is shared by glaucophytes and chromalveolates (contig 2035b.17, Fig. 2c ) and another that is shared only by red algae (contig 2035b.28, Fig. 2d ). To gain a broader perspective on E/HGT, we also inspected phylogenies associated with all carbohydrate-active enzymes (CAZymes) identified in P. purpureum (see below for details). This revealed that of 107 CAZyme trees that could be interpreted with respect to prokaryotic or eukaryotic origin of the gene in P. purpureum , 41 genes (38%) had a prokaryotic provenance. Some of these genes were limited to red algae, whereas others were shared solely with Plantae and many (25 genes) had spread to chromalveolates. 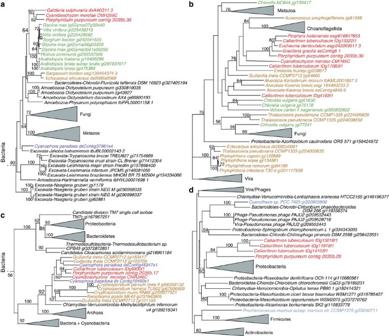Figure 2: Phylogenetic analysis of proteins on contig 2035b inP. purpureum. These are all RAxML trees (WAG + Γ + I + F model) with the results of 100 bootstrap replicates shown on the branches. (a) Tree inferred from a squalene monooxygenase-like protein involved in sterol biosynthesis that shows the expected monophyly of red algae and of plants within the eukaryote tree of life. (b) Tree inferred from a tyrosine kinase/lipopolysaccharide-modifying enzyme that shows a complex phylogenetic relationship between red algae and chromalveolates. (c) Tree inferred from a glycosyltransferase of bacterial origin that is consistent with the monophyly of red algae and glaucophytes and a shared history of the gene in these taxa with chromalveolates, potentiallyviasecondary EGT. (d) Tree inferred from an unknown protein in the aminotransferase superfamily that is present only in red algae and originated through HGT presumably from a proteobacterial source. The unit of branch length in each tree is the number of substitutions per site. The GenBank GI and Joint Genome Institute (JGI) accession codes (where available) are shown after each taxon name. Figure 2: Phylogenetic analysis of proteins on contig 2035b in P. purpureum . These are all RAxML trees (WAG + Γ + I + F model) with the results of 100 bootstrap replicates shown on the branches. ( a ) Tree inferred from a squalene monooxygenase-like protein involved in sterol biosynthesis that shows the expected monophyly of red algae and of plants within the eukaryote tree of life. ( b ) Tree inferred from a tyrosine kinase/lipopolysaccharide-modifying enzyme that shows a complex phylogenetic relationship between red algae and chromalveolates. ( c ) Tree inferred from a glycosyltransferase of bacterial origin that is consistent with the monophyly of red algae and glaucophytes and a shared history of the gene in these taxa with chromalveolates, potentially via secondary EGT. ( d ) Tree inferred from an unknown protein in the aminotransferase superfamily that is present only in red algae and originated through HGT presumably from a proteobacterial source. The unit of branch length in each tree is the number of substitutions per site. The GenBank GI and Joint Genome Institute (JGI) accession codes (where available) are shown after each taxon name. Full size image Light-harvesting complex proteins in P. purpureum Cyanobacteria and algae use light-harvesting proteins that contain photopigments to channel the energy gained from photons toward the chlorophyll-containing reaction centres of photosystems PSI and PSII. In many cyanobacteria, the only light-harvesting antenna proteins are phycobilisomes. In green algae and plants, all light-harvesting proteins are members of the light-harvesting complex (LHC) family [21] . In contrast, red algae are an intermediate between the two because they contain phycobilisomes, primarily associated with PSII, while also containing LHC proteins associated with PSI. P. purpureum was the first organism to have its phycobilisomes isolated and some of the phycobiliproteins (PBPs) and the LHC proteins have been characterized [22] . We identified seven LHC proteins in the P. purpureum genome (contigs 435.19, 491.7, 776.1, 2142.1, 2493.3, 3421.1 and 4406.7; see Supplementary Fig. S6A ), which is consistent with previous analyses [21] . The sequence encoded on contig 491.7 was identical to the previously identified Lhcr1 from P. purpureum and the sequence encoded on contig 2493.3 was identical to Lhcr2 (refs 23 , 24 ). The other five LHC proteins were compared with the N-terminal fragment data from Tan et al . [23] ( Table 2 ). Whereas these authors identified six unique protein bands, their sequencing results suggested that the 19.5 kDa band contained two unique proteins, which our results confirm [23] . Therefore, all seven P. purpureum LHC proteins are expressed. Phylogenetic analysis of the LHC proteins showed that, as expected, the P. purpureum sequences grouped with other red algae and chromalveolates ( Supplementary Fig. S6A ). Table 2 Comparison of molecular weights based on sequence prediction. Full size table Analysis of phycobilisome proteins showed P. purpureum contains alpha and beta subunits for phycoerythrin (PE) as well as several linker proteins (including L CM , L RC , L C and 4 γ PE ) (see Supplementary Data 1 ). Surprisingly, we found a nuclear-encoded alpha-like PBP ( Supplementary Fig. S6B ). As PBP bands are not well resolved in SDS–PAGE gels [25] , it is difficult to estimate from previous research the number of PBPs expressed in P. purpureum . The novel protein encoded on contig 2051.9 (252 aa in length) is associated in the tree with a number of cyanobacterial genes, one of which is a second α AP (allophycocyanin) from Gloeobacter violaceus (gi37520823). Whereas this second AP-α protein was identified from the sequencing of the G. violaceus genome [26] , analysis of the phycobilisomes did not identify any homologues in P. purpureum to the gi37520823 gene product. Examination of the G. violaceus genome shows this gene to be in an apparent operon with a bilin biosynthesis protein (MpeU-like protein) and a hypothetical protein, suggesting that if expressed it likely has a role in light harvesting (results not shown). The transcriptome data from P. purpureum shows extensive expression (813 mapped reads) of the novel PBP-encoding gene and examination of the protein sequence reveals a ca. 60 amino acid N-terminal extension when compared with cyanobacterial homologues. This extension appears to specify plastid targeting (scores of TargetP=0.65, ChloroP=0.67, Predotar=0.26 and Wolfpsort=14.0) and contains a phenylalanine near the N-terminus (that is, in this case, MLMFVF) that is typical for Plantae plastid targeted proteins [5] . Although lacking introns (as do most P. purpureum genes), these data suggest the red algal gene is a nuclear-encoded plastid-targeted PBP. A phylogenetic tree that includes all of the PBPs and core-membrane linkers ( Supplementary Fig. S7 ) demonstrates the evolutionary relationship between the alpha and beta subunits and AP, PC, PE and the core-membrane linker and is consistent with previous data [27] . 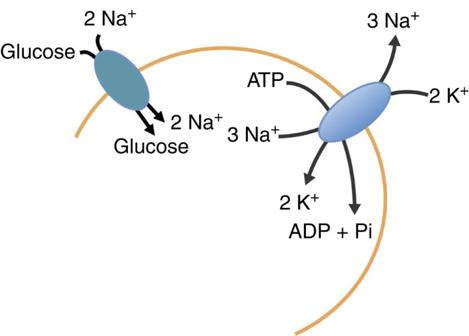Figure 3: Analysis of a transporter inP. purpureum. Schematic image showing the putative sodium–potassium ATPase and sodium:glucose cotransporter identified in theP. purpureumgenome data. Analysis of CAZymes and starch biosynthesis A total of 116 putative CAZymes and 40 additional proteins containing putative carbohydrate-binding modules were identified in P. purpureum ( Table 3 ) using the CAZy annotation pipeline [28] . These genes have a complex phylogenetic history ( Supplementary Tables S10–S12 ). The genome of P. purpureum encodes 31 glycoside hydrolases (GH), 83 glycosyltransferases (GT) and two carbohydrate esterases, but similar to other unicellular rhodophytes and chlorophytes, lacks homologues of known polysaccharide lyases. P. purpureum encodes a larger number of GH and GT (114) genes when compared with C. merolae (82). Not surprisingly, the number of CAZy families is also 33% greater in P. purpureum (14 GH and 34 GT families) when compared with C. merolae (9 GH and 27 GT families), likely reflecting the complexity of P. purpureum cell-wall polysaccharides [29] . In comparison with the highly complex pathways of starch metabolism in green algae (over 30 genes) and the more diverse pathway in glaucophytes (22 genes), P. purpureum displays an unusually simple enzyme network consisting of 19 genes with many critical biosynthetic steps represented by single enzymes. This includes a single soluble starch synthase (GT5) that must have the remarkable property of priming polysaccharide synthesis, seeding the formation of novel granules and elongating the different size classes of chains present on amylopectin. These functions require a minimum of four distinct types of enzymes in Viridiplantae and several analogous glucan synthases in glaucophytes [30] . More exceptional and seemingly not shared with other starch accumulating red algae is the likely presence of a single isoamylase gene (contig 3410.5). Distinct isoamylase-like GH13 glycoside hydrolases are known to be involved both in starch catabolism and in the synthesis of the amylopectin crystalline structure that distinguishes starch from glycogen. This dual function seems to require several isoamylase genes in all Plantae examined thus far [30] . The presence of this single enzyme brings into question its involvement in both processes. However, absence of a second isoamylase correlates with the presence of three GH13 α-amylase candidate sequences. One of these (contig 4541.5) may have debranching activity [31] . This GH13 glycoside hydrolase is also found in some starch accumulating algae that apparently lack isoamylase genes and have a red algal plastid derived from secondary endosymbiosis. Of great interest here is the presence of another α-glucan synthase encoding gene ( GT5 ), a granule-bound starch synthase that correlates with the presence of amylose in Porphyridiales ( Porphyridium or Rhodella ) [32] , a unique feature of these unicellular algae when compared with other Rhodophyta. Other aspects of carbohydrate metabolism in P. purpureum are presented in the Supplementary Information . Table 3 CAZymes present in the P. purpureum genome. Full size table Membrane transporters in P. purpureum About 3.4% of the 8,355 predicted genes in the P. purpureum genome encode solute transporters, channels and pumps, which is similar to the corresponding numbers in green algae and land plants ( Supplementary Data 2 ). Strikingly, in contrast to the currently known genomes of land plants and green and red algae, P. purpureum contains a putative sodium–potassium ATPase (encoded on contig 2281.11). Sodium–potassium ATPases import K + into cells and Na + out of cells at the expense of ATP, thereby keeping intracellular sodium concentrations low and potassium concentrations high ( Fig. 3 ). Thus, the pump contributes to maintaining cellular potassium and sodium homoeostasis in P. purpureum , which is exposed to high extracellular sodium concentrations in its environment. Furthermore, the sodium gradient across the plasma membrane that is set up by the sodium–potassium pump provides the driving force for secondary active sodium-coupled solute transporters. Indeed, the P. purpureum genome encodes several putatively sodium-driven transporters, such as a sodium:bicarbonate symporter (contig 2098.9), a sodium-dependent phosphate transport system (contig 2023.2), and a sodium:glucose cotransporter ( Fig. 3 ), which is the first finding of a such a transporter in a photosynthetic organism. Interestingly, it has been recently demonstrated that P. purpureum can be grown to high cell densities in complete darkness with glucose as the sole carbon source [33] . In addition to the sodium:glucose symporter, four putative sucrose transporters were found in P. purpureum (contigs 2016.15, 2025.48, 2077.1, 3677.2). Among photosynthetic eukaryotes, sucrose transporters until now have only been reported from land plants and from the extremophilic red alga Galdieria sulphuraria that is able to grow heterotrophically on a range of different carbon sources [34] . It is thus possible that P. purpureum in addition to the monosaccharide glucose is also able to exploit disaccharides, such as sucrose, for heterotrophic growth, likely by a proton-coupled co-transport mechanism. Alternatively, because genes encoding the enzymes required for sucrose catabolism are not detectable in the P. purpureum genome (see Supplementary Methods ), these transporters might be involved in the transport of osmotically active solutes, such as trehalose or mannosylglycerate. Figure 3: Analysis of a transporter in P. purpureum. Schematic image showing the putative sodium–potassium ATPase and sodium:glucose cotransporter identified in the P. purpureum genome data. Full size image Cytochrome P450 genes in P. purpureum Cytochrome P450 (CYP) is one of the largest gene families with 5,100 sequences annotated in plants, 1,461 in vertebrates, 2,137 in insects, 2,960 in fungi, 1,042 in bacteria, 27 in Archaea and two in viruses [35] . Red algae are characterized by small genome sizes and therefore the species sequenced until now have a small number of CYP genes compared with Viridiplantae. The P. purpureum nuclear genome encodes 12 CYP genes ( Supplementary Table S13 ), whereas C. merolae and G. sulphuraria contain 5 and 7 CYP genes, respectively. The P. purpureum CYPs contain all the conserved P450 domains ( Supplementary Table S14 ), however, only three of these genes are orthologs of CYP clades already described: contig 3544.1 (CYP97), contig 2697.2 (CYP51) and contig 440.7 (CYP710). The remaining 9 CYP genes group with diverse eukaryotes in novel clades ( Fig. 4a ). Other aspects of CYP evolution in P. purpureum are presented in the Supplementary Information . 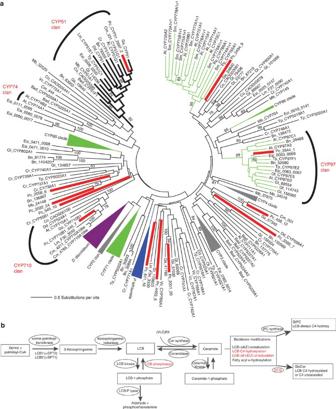Figure 4: Analysis of CYPs and sphingolipid metabolism inP. purpureum. (a) Maximum likelihood (RAxML; LG + Γ + I + F model) tree of CYP sequences fromP. purpureumand other eukaryotes. Support for internal branches was assessed using 100 bootstrap replicates. The major known CYP clans are indicated. (b) Putative sphingolipid synthesis pathway inP. purpureumdeduced from analyses of vascular plants (for example,Arabidopsis). Modifications without candidate genes in theP. purpureumdraft assembly are indicated in red. Cer, ceramide; GCS, glucosylceramide synthase; GIPC, glucosyl inositol phosphoryl ceramide; GlcCer, glucosylceramide; IPC, inositol phosphoryl ceramide; LCB, long chain base; and VLCFA, very long chain fatty acid. Figure 4: Analysis of CYPs and sphingolipid metabolism in P. purpureum . ( a ) Maximum likelihood (RAxML; LG + Γ + I + F model) tree of CYP sequences from P. purpureum and other eukaryotes. Support for internal branches was assessed using 100 bootstrap replicates. The major known CYP clans are indicated. ( b ) Putative sphingolipid synthesis pathway in P. purpureum deduced from analyses of vascular plants (for example, Arabidopsis ). Modifications without candidate genes in the P. purpureum draft assembly are indicated in red. Cer, ceramide; GCS, glucosylceramide synthase; GIPC, glucosyl inositol phosphoryl ceramide; GlcCer, glucosylceramide; IPC, inositol phosphoryl ceramide; LCB, long chain base; and VLCFA, very long chain fatty acid. Full size image Glycerolipid biosynthesis Membrane glycerolipid biosynthesis in P. purpureum follows the same path as is present in vascular plants and red algae such as Porphyra [17] or C. merolae [36] but with a few minor differences. In line with findings from other red algae, genes encoding the acetyl-CoA carboxylase subunits ( accA , accB and accD ) are encoded in the plastid, not the nuclear genome, as is the case for members of the Viridiplantae and their derived secondary endosymbionts. As also described for other red algae [17] , [36] , P. purpureum lacks a plastid desaturation pathway including the gene encoding the soluble stearoyl acyl-ACP desaturase ( FAB2 ) present in all members of the green lineage. This indicates that saturated C 16 – and C 18 – rather than monounsaturated fatty acids are exported from the plastid to the endoplasmic reticulum (ER). The first step in the biosynthesis of polyunsaturated fatty acids is catalysed by a Δ9-desaturase. The protein sequence encoded on contig 2306.6 contains an N-terminal cytochrome b 5 domain, distantly related versions of which are present in red algae and fungi, but absent in plants. P. purpureum is able to synthesize eicosapentaenoic acid (EPA, 20:5 Δ [5] , [8] , [11] , [14] , [17] ). All required enzymes are encoded as single-copy genes in the nucleus and likely located in the ER with one exception. For the putative ω3-desaturase encoded on contig 2141.6 that catalyses the last step of EPA biosynthesis, a putative plastid transit peptide was identified and as expected, the N-terminus of the protein encoded phenylalanine residues (that is, MFAGF), indicating that ω3-desaturation takes place inside this organelle. This is in line with observations from labelling experiments [37] but contrasts with analyses of Porphyra EST data [17] . In contrast to findings in other red algae, some genes involved in glycerolipid synthesis appear to be present in multiple copies. Three candidate genes encoding monogalactosyl diacylglycerol transferase (MGD) and two genes encoding digalactosyl diacylglycerol transferase (DGD) homologues required for galactolipid synthesis were identified. The model plant Arabidopsis thaliana also contains three MGD and two DGD orthologs. Whereas MGD1 and DGD1 are constitutively active at the chloroplast inner envelope, MGD2, MGD3 and DGD2 are present at the chloroplast outer envelope following phosphate deprivation. Under these conditions, phospholipids in ER membranes are replaced by galactolipids. This phenomenon is also known from other organisms including some bacteria, but remains to be biochemically validated in P. purpureum . Synthesis of sphingolipids Sphingolipids are ubiquitous lipids that are highly enriched in the plasma membrane [38] . They are composed of an amino alcohol, the so-called sphingoid (long chain) base, amide-linked to a fatty acid. The long chain base can be further modified by the addition of complex sugar headgroups. Apart from their function as membrane building blocks, some sphingolipids also have signalling functions and are, for example, involved in cell cycle control and programmed cell death [39] . We identified all genes necessary for the formation of complex glycosphingolipids in the nuclear genome of P. purpureum ( Fig. 4b and Supplementary Table S15 ). In addition to the findings in the Porphyra transcriptome [17] , we also found a candidate for a long chain base-kinase (contig 4419.4). Unlike protein sequences from Viridiplantae, the candidate for the fatty acid α-hydroxylase (encoded on contig 522.16) contains an N-terminal cytochrome b 5 domain similar to that in fungal orthologs. Possible evidence of sexual reproduction in P. purpureum Multicellular red algae within the Florideophyceae are well known for their complex triphasic life cycles. Sexual reproduction is also known in Bangiophyceae such as Porphyra that has a haploid gametophyte and a diploid ‘conchocelis’ stage [40] . Interestingly, one of the oldest multicellular eukaryotic fossils is believed to be the gametophytic stage of a Bangiophyceae, dating to rocks up to 1,200 million years old [41] . Outside of the Florideophyceae and Bangiophyceae, however, very little is known about sexual reproduction in red algae, particularly for unicellular forms such as P. purpureum , with most accounts suggesting the lack of sex in this lineage [42] . This is surprising because sexual reproduction is believed to be an ancient feature of eukaryotes [43] , [44] and relatively few lineages have completely lost this ability. To address the possibility of ‘cryptic sex,’ we searched the P. purpureum genome for the eight meiosis-specific proteins SPO11, HOP1, HOP2, MND1, DMC1, MSH4, MSH5, REC8 and MER3 (ref. 45 ). The presence of genes encoding a majority of these proteins is taken as evidence for meiosis and therefore sexual reproduction (for example, in Giardia intestinalis [43] , Trichomonas vaginalis [45] ). Our search turned up evidence for eight of the targeted proteins ( Table 4 ) including two paralogs of SPO11 (SPO11-2 and SPO11-3). All trees are shown in Supplementary Figs S8–S15 . The presence of 8 out of 9 meiosis-specific proteins is consistent with (but does not prove) the maintenance of sexual reproduction in P. purpureum . Presence of all ‘toolkit’ proteins is not required for sexual reproduction. There are numerous examples of species known to be sexual that are missing one or more of these proteins. For example, Drosophila melanogaster lacks DMC1, HOP2, MND1, MSH4 and MSH5 (ref. 44 ). It would not be unusual if P. purpureum lacks REC8, because most protists, including known sexual species such as Chlamydomonas , also do not have this protein [44] . It is likely that in lineages missing REC8, RAD21 (the mitotic paralog) functions as well in meiosis. In the case of P. purpureum , the two identified contigs could be the result of a RAD21 gene duplication, whereby one of the paralogs has assumed a meiotic function. Table 4 Identification of the meiotic toolkit genes in P. purpureum . Full size table Analysis of the first genome sequence from a mesophilic, unicellular red alga turned up several surprises. First, the genome is tightly packed with coding regions and is intron poor, reminiscent of a bacterial genome. There are very few large gene families, suggesting that unicellular red algal extremophiles and mesophiles may have undergone a phase of genome reduction, perhaps in an extremophilic common ancestor of all Rhodophyta. It is also interesting (if not surprising) that hundreds (5.4–9.3%) of the 8,355 P. purpureum genes show evidence of a reticulated evolutionary history and are likely to be implicated in E/HGT, with many more gene with phylogenies that cannot be readily interpreted using existing data. These data shed light on recent debates about the role of HGT in microbial eukaryote genome evolution, in particular whether phagotrophic and parasitic lineages are more likely to capture foreign genes than strict photoautotrophs [46] , [47] . In contrast to expectations, we demonstrate that anciently diverged relatives of the free-living, photosynthetic P. purpureum were mediators of HGT between prokaryotes and photosynthetic eukaryotes, vis-à-vis endosymbiosis. We have, however, no way of knowing for certain whether the red algal (or Plantae) ancestor was phagotrophic and therefore more prone to HGT, because evidence of HGT has also been described in non-phagotrophic lineages [48] . Regardless of the mechanism of ancient or more recent HGT, these data underline the fundamental importance of red algae to the evolution of eukaryotic plankton. Red algal plastids and red algal nuclear genes are now widespread in chlorophyll c -containing lineages such as diatoms, haptophytes and cryptophytes. Other highlights of this genome include the finding of a nuclear-encoded PBP that apparently has a plastid function (that is, supported by the presence of a putative plastid-targeting signal), an unexpected diversity of CYP genes compared with green plants, and a simpler pathway for starch biosynthesis (see Supplementary Data 3 for a list of the plastid encoded genes). As red algae have the longest fossil record known among eukaryotes (1.2 billion years [41] ) and the lineage contains up to 14,000 species [1] , P. purpureum provides promise that a wealth of novel information awaits to be unearthed as additional genomes are completed from Rhodophyta. Genome sequencing A total of 7.4 Gbp of P. purpureum CCMP 1328 paired end (150 × 150 bp) genome data generated using two flow cell lanes in the Illumina GAIIx were assembled with the CLC Genomics Workbench tools ( http://www.clcbio.com/products/clc-genomics-workbench/ ) into 4,770 contigs with a N50 of 20,296 bp. The contigs had average nucleotide coverage of 376 × (median=56 × ) and totalled 19.7 Mbp, suggesting a genome size of ca. 20 Mbp. As with other genome studies, these estimates are subjected to further validation with better assembly of more sequence data. Thereafter, 4.1 Gbp of Illumina mRNA-seq data (150 bp x 150 bp reads) were used to train the ab-initio gene predictors (for details, see Price et al . [5] ), resulting in a set of 8,355 weighted consensus gene structures that were used for downstream analyses. Genome-wide analysis and phylogenomics Repeat elements were identified using RepeatMasker ( http://www.repeatmasker.org/ ) against the Repbase repetitive DNA elements library (version 2012-04-18) and a de novo repeat library elements generated using Repeat modeller ( http://www.repeatmasker.org/ ). Duplicated genes from red algal genomes were identified using the method described in a previous study [49] , except that we required aligned regions to cover >70% length of both proteins of the duplicated genes. The identity ( I ) cutoff for paralogous gene pairs was 30% if the total length of the aligned regions ( L ) was >150 amino acids. When L was ≤150 amino acids, then the minimal I was found [50] using the formula I ≥0.06+4.8 L −0.32(1+ exp(− L /1,000)) . Paralogous gene pairs were clustered into gene families. A gene was assigned to a gene family if it was paralogous to one or more of its members. Phylogenomic analysis was done based on protein sequence alignments as previously described [4] , [5] using MUSCLE 3.8.31 (ref. 51 ) (default settings) and RAxML 7.2.8 (ref. 52 ) (WAG + Γ model; 100 bootstrap replicates). Only trees that contained ≥3 phyla and a minimum number of taxa ( N ) ranging from 4 to 40 were considered, to minimize the impact of taxon sampling on this analysis. The screening for gene transfer is based on strongly supported clades consisting of rhodophyte(s) and one other phylum, as described in an earlier study [53] , where prokaryote (or when unavailable, opisthokont) sequences were used as outgroup in rooting the trees. A phylogenetic tree was considered to show non-exclusive sharing of a Plantae gene when a strongly supported clade (at the defined bootstrap support threshold) was found that comprised ≥90% Plantae taxa with the remainder being non-Plantae (for example, stramenopiles). This type of gene history implies putative E/HGT between the Plantae and non-Plantae taxa, but nevertheless provides support for Plantae monophyly. We did not interpret these trees as evidence of E/HGT. Analysis of gene functional biases Based on the annotated GO terms ( http://geneontology.org/ ) using Blast2GO [19] (BLASTp E ≤10 −5 ), we applied Fisher’s exact test to assess potential functional biases in a given set of P. purpureum genes (test set; for example, genes associated with Plantae or non-Plantae taxa) in comparison with the annotated terms across the overall 8,355 genes (the reference set; see Supplementary Tables S7–S9 ), with correction for multiple testing [54] . An over- or under-representation of a GO term in the test set is statistically significant when P ≤0.05 and false discovery rate ≤0.10. Identification and bioinformatic analysis of CAZymes All 8,355 putative ORFs encoded by the P. purpureum genome were submitted to analysis using the CAZy annotation pipeline in a two-step procedure of identification and annotation [28] . Sequences were subjected to BLASTp analysis against a library composed of the full-length proteins of the CAZy database. The hits with an e -value better than 0.1 were then subjected to a modular annotation procedure, that combines BLASTp against libraries of catalytic and carbohydrate-binding modules and family-specific profile Hidden Markov models (for details, see Price et al . [5] ). The results were manually verified and completed with signal peptide, transmembrane and GPI predictions [55] , [56] . The fragmentary models and all models suspected of prediction errors were identified and flagged. Finally, a functional annotation step was carried out involving BLASTp comparisons against a library of modules derived from biochemically characterized enzymes [28] . Analysis of CYP genes The P. purpureum protein models were searched by BLASTp analysis with CYP protein sequences representing the CYP2, CYP3 and CYP4 animal clades [57] , and the CYP51,CYP71, CYP72, CYP74, CYP85, CYP86, CYP97, CYP710, CYP711, CYP727 and CYP746 plant clades [35] . P450 sequences from other species, including those from Bigelowiella natans and Guillardia theta [58] , were identified in the same way and their CYP denomination were confirmed whenever possible using the standard P450 classification [59] . Their CYP sequences accession codes and provenances are summarized in Supplementary Table S13 . The distantly related clade CYP727 and the divergent sequences CYP804A1 and CYP772A1 were excluded from the phylogenetic analysis. The CYP sequences were aligned using MUSCLE 3.8.31 (ref. 51 ) and a tree constructed using RAxML [52] (WAG + Γ + I model; 100 bootstrap replicates). Microscopy Transmission electron microscopy images were taken at the Center of Advanced Microscopy at Michigan State University, East Lansing, MI, USA on a JEOL100 CXII instrument (Japan Electron Optics Laboratories, Tokyo, Japan). For sample preparation, P. purpureum CCMP 1328 cells were processed as previously described [60] . Accession codes: Coordinates for the draft P. purpureum genome and the Illumina mRNA-seq reads from this alga have been deposited at the NCBI Sequence Read Archive (SRA) with Project number BioProject ID# PRJNA189757 , under the accession code SRP018727 . How to cite this article: Bhattacharya, D. et al . Genome of the red alga Porphyridium purpureum . Nat. Commun. 4:1941 doi: 10.1038/ncomms2931 (2013).